Transition to a Bose–Einstein condensate and relaxation explosion of excitons at sub-Kelvin temperatures Quasiparticles in quantum many-body systems have essential roles in modern physical problems. Bose–Einstein condensation (BEC) of excitons in semiconductors is one of the unobserved quantum statistical phenomena predicted in the photoexcited quasiparticles in many-body electrons. In particular, para-excitons in cuprous oxide have been studied for decades because the decoupling from the radiation field makes the coherent ensemble a purely matter-like wave. However, BEC has turned out to be hard to realize at superfluid liquid helium-4 temperatures due to a two-body inelastic collision process. It is therefore essential to set a lower critical density by further lowering the exciton temperature. Here we cool excitons to sub-Kelvin temperature and spatially confine them to realize the critical number for BEC. We show that BEC manifests itself as a relaxation explosion as has been discussed in atomic hydrogen. The results indicate that dilute excitons are purely bosonic and BEC indeed occurs. Bose–Einstein condensation (BEC) is a quantum mechanical phenomenon directly linked to the quantum statistics of bosons. While cold atomic gases provide a new arena for exploring the nature of BEC [1] , [2] , [3] , [4] , a long-term quest to confirm BEC of excitons, quasi-Bose particles formed as a bound state of an electron-hole pair, has been underway since its theoretical prediction in the 1960s [5] , [6] . Ensembles of electrons and holes are complex quantum systems with strong Coulomb correlations; thus, it is non-trivial whether nature chooses a form of exciton BEC. Various systems have been examined in bulk [7] , [8] , [9] and two-dimensional semiconductors [10] , [11] and also in exciton–photon hybrid systems [12] , [13] , [14] . Among them, the 1 s paraexciton state in a single crystal of Cu 2 O has been a prime candidate for realizing spontaneous build up of a three-dimensional BEC that is decoupled from radiation field. The large binding energy and long lifetime enable the preparation of cold excitons in thermal equilibrium with the lattice. However, collisional loss [15] , [16] severely limits the conditions for reaching BEC. Such a system with a large inelastic cross-section is excluded in atomic BEC experiments, where a small inelastic scattering rate and efficient elastic scattering are necessary for evaporative cooling. Here we demonstrate that it is nevertheless possible to achieve BEC by cooling paraexcitons to sub-Kelvin temperatures in a cold phonon bath. Emission spectra from paraexcitons in a three-dimensional trap show an anomalous distribution in a threshold-like manner at the critical number of BEC expected for ideal bosons. This phenomenon in the external potential can be understood as a relaxation explosion that is discussed in atomic BECs with small elastic scattering lengths and considerable inelastic scattering processes. Bosonic stimulated scattering into the condensate and the collisional loss compete and limit the condensate to a fraction of about 1%. This observation adds a new class of experimentally accessible BEC and provides us opportunities for exploring a rich variety of matter phases of electron-hole ensembles. Properties of paraexcitons The 1 s paraexciton is the pure spin triplet state, so it is decoupled from the radiation field. In high-quality single crystals, excitons show very long lifetimes of more than hundreds of nanoseconds [16] , [17] , reaching thermal equilibrium with the lattice. The corpuscular nature of excitons is well visualized in emission spectra reflecting their thermal distribution. As paraexcitons are light quasi-particles (effective mass m ex =2.6 m 0 ( m 0 is the electron mass at rest) [18] ), BEC has been believed to be attainable at moderate density ( n ∼ 10 17 cm −3 ) at the temperature of superfluid helium (2 K) (refs 7 , 8 , 9 ). However, a two-body inelastic collision process that hampers efficient accumulation and cooling prevents the realization of exciton BEC in Cu 2 O [15] . A recent paraexciton density evaluation with a wide dynamic range [16] showed that rather dilute ( n ∼ 10 14 cm −3 ) paraexcitons increase sublinearly with the excitation rate, so that the crystal (and excitons) should suffer significant heating in achieving a density of 10 17 cm −3 . This effect is well known as an efficient collision-induced loss channel for 1 s orthoexcitons (the second-lowest exciton level, with lifetimes of a few ns) [15] . Scattering cross-sections In atomic BEC experiments [1] , [2] , [3] , [4] , [19] , s -wave elastic scattering cross-sections (or equivalently, scattering lengths) are crucial parameters. The elastic scattering cross-section σ el should be significantly larger than the inelastic cross-section σ inel to obtain a quantum degenerate gas via efficient evaporative cooling. Only the atomic species that fulfil this condition are preselected. Despite the importance of scattering properties, little information on the scattering cross-section of paraexcitons has been obtained until recently. We summarize the characteristics of the 1 s exciton in Cu 2 O, whose Bohr radius is about 0.7 nm. When the temperature is lowered, the inelastic cross-section diverges (that is, the two-body collision-induced loss coefficient does not depend on temperature). Such behaviour is typical of quantum-mechanical inelastic collisions and is known as the inverse velocity law of s -wave inelastic scattering [20] . The measured value (with a factor of three in error) for paraexcitons is σ inel =85 nm 2 at 5 K (ref. 16 ). From the inelastic cross-section, we estimate an elastic cross-section of 23≤ σ el ≤85 nm 2 ( Supplementary Information ); quantum Monte Carlo calculations [21] show σ el =50 nm 2 . As the inelastic cross-section is inversely proportional to the square root of the temperature, and the elastic cross-section is temperature independent, the inelastic collisional loss rate is always at the same level or higher than the elastic scattering rate and therefore governs the properties of the system at low temperature. To achieve BEC, we must set the critical density as low as possible by lowering the exciton temperature to circumvent the collision-induced loss. Inefficient elastic collisions cannot redistribute the excess energy generated in inelastic collisions. However, in solid-state systems, a phonon bath ensures the thermal equilibrium of the excitons. In principle, BEC is possible even when inelastic collisions dominate. Such a situation is inaccessible in atomic experiments, and thus the present system can offer a unique opportunity to study a new type of BEC. Trapping paraexcitons at sub-Kelvin temperatures We use a 3 He refrigerator to cool the crystal as low as 278 mK. To avoid ballistic diffusion of excitons [22] and to accumulate excitons under quasi-continuous-wave (cw) feeding, we prepare a three-dimensional harmonic potential trap with an inhomogeneous applied strain [23] , [24] (Methods). We design a sample holder with a built-in spring that blocks any incoming heat to apply static pressure to the crystal. The trap frequencies in the xy and z -directions ( Fig. 1a ) are ω x,y =2π×17 MHz and ω z =2π×25 MHz, respectively ( Supplementary Information ), to be compared with the lifetime of 300 ns ( Supplementary Information ). The excitation cw laser incoherently generates 1 s orthoexcitons (12 meV above the 1 s paraexciton level) via a phonon-assisted absorption process in a cigar-shaped volume around the bottom of the trap ( Fig. 1b,c ). The orthoexcitons convert into 1 s paraexcitons in nanoseconds and subsequently flow towards the bottom of the trap potential. Paraexcitons release their excess kinetic energy to the phonon bath via scattering with acoustic phonons on their way to the bottom; thus, sufficiently cold paraexcitons accumulate near the potential minima. We detected spatially resolved, time-integrated luminescence spectra of direct radiative recombination of paraexcitons, which is slightly allowed by the strain field [25] . 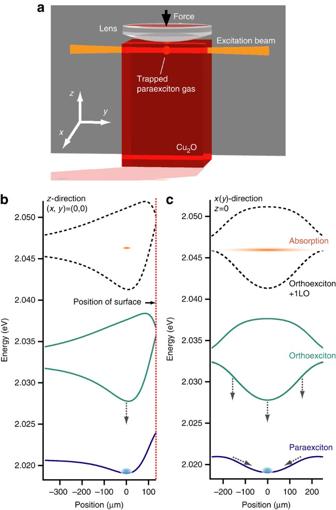Figure 1: Capturing cold 1sparaexcitons in a single Cu2O crystal. (a) Inhomogeneous strain field is formed by pressing the single crystal with a glass lens. The field acts as a three-dimensional harmonic trap for paraexcitons, where the trap bottom is located 133 μm below the surface of the crystal. A focused excitation laser beam passes through the bottom of the trap. (b,c) The strain field causes a position-dependent energy shift for both ortho- and paraexcitons. The excitation beam creates orthoexcitons only around the trap via a phonon-assisted absorption process; they rapidly convert to paraexcitons with their position almost unchanged. Paraexcitons flow into the bottom of the trap, dissipating their excess energy to the lattice. Accumulated paraexcitons move along the trap potential coherently owing to the very small interaction rate of cold paraexcitons with phonons. Figure 1: Capturing cold 1 s paraexcitons in a single Cu 2 O crystal. ( a ) Inhomogeneous strain field is formed by pressing the single crystal with a glass lens. The field acts as a three-dimensional harmonic trap for paraexcitons, where the trap bottom is located 133 μm below the surface of the crystal. A focused excitation laser beam passes through the bottom of the trap. ( b , c ) The strain field causes a position-dependent energy shift for both ortho- and paraexcitons. The excitation beam creates orthoexcitons only around the trap via a phonon-assisted absorption process; they rapidly convert to paraexcitons with their position almost unchanged. Paraexcitons flow into the bottom of the trap, dissipating their excess energy to the lattice. Accumulated paraexcitons move along the trap potential coherently owing to the very small interaction rate of cold paraexcitons with phonons. Full size image Temperature of paraexcitons First, we examined the temperature dependence of the signal ( Fig. 2a–c ) under low-density excitation (3×10 6 paraexcitons in the trap at the lowest temperature), where density-dependent processes are negligible. Above 1 K, the size of the cloud ( Fig. 2d ) and the spectral width ( Fig. 2e ) coincide perfectly with a theoretical prediction assuming the classical thermal distribution (modified for direct luminescence in the strain-induced harmonic potential [23] ). This ensures that the exciton gas is in thermal equilibrium with the lattice. However, at T L ≤1 K, the exciton temperature remains higher than that of the lattice, indicating that exciton cooling by phonon emission becomes inefficient; namely, the exciton–phonon scattering time becomes comparable to or longer than the exciton lifetime. From the spatial and spectral widths, the temperature of the exciton gas stays at T =0.8 K when T L ≤0.6 K. The critical number for BEC of non-interacting Bose gas at T =0.8 K is N c =7.6×10 8 from the equation where ς ( x ) and denote the Riemann zeta function and geometric average of the angular frequency respectively. The increase in integrated intensity ( Fig. 2f ) at lower T L reflects the increased capture efficiency of the trap and increased emission collection of the shrunken cloud image on the entrance slit of the spectrometer (7.5 μm wide on the cloud). 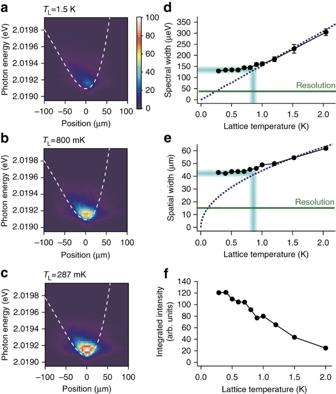Figure 2: Coherent trapping of 1sparaexcitons at sub-Kelvin lattice temperatures. Trapped paraexciton gas is observed via direct luminescence, which is only weakly allowed under the applied strain field. The spatially resolved luminescence is recorded as a function ofTLunder the weakest excitation condition. (a)TL=1.5 K. (b)TL=800 mK. (c)TL=287 mK. Dashed curves are calculated potential profiles of the harmonic trap. (d–f) Spatial full width at half maximum (FWHM), spectral FWHM and total luminescence intensity of the paraexciton gas along thez-axis, respectively, versus the lattice temperature. Dashed curves are theoretical predictions assuming the classical thermal distribution. Green lines show experimental resolution of our setup. Figure 2: Coherent trapping of 1 s paraexcitons at sub-Kelvin lattice temperatures. Trapped paraexciton gas is observed via direct luminescence, which is only weakly allowed under the applied strain field. The spatially resolved luminescence is recorded as a function of T L under the weakest excitation condition. ( a ) T L =1.5 K. ( b ) T L =800 mK. ( c ) T L =287 mK. Dashed curves are calculated potential profiles of the harmonic trap. ( d–f ) Spatial full width at half maximum (FWHM), spectral FWHM and total luminescence intensity of the paraexciton gas along the z -axis, respectively, versus the lattice temperature. Dashed curves are theoretical predictions assuming the classical thermal distribution. Green lines show experimental resolution of our setup. Full size image Note that two distinct features are needed to pursue paraexciton BEC at sub-Kelvin temperatures. The first is coherent harmonic motion of paraexcitons in a trap. To establish the energy structure of excitons in a three-dimensional harmonic potential trap, their mean scattering time should be longer than the period of harmonic oscillation. Therefore, the exciton–phonon scattering rate (Γ phonon ) must be less than the trap frequency ( f trap ): Γ phonon < f trap . This has not been realized in previous trap experiments at liquid 4 He temperatures, where Γ phonon is a few hundred MHz and f trap is 13 MHz [23] . At sub-Kelvin temperatures, the phonon scattering time is reduced and is comparable to the exciton lifetime of 300 ns ( Supplementary Information ). This implies that Γ phonon is a few MHz, which satisfies the condition described above. The second is smaller heating resulting from weaker excitation power. Owing to the large σ inel , the collision-limited paraexciton number N effectively scales as N ∝ G 0.5 , where G is the generation rate of excitons or the optical excitation power. Because the exciton gas is captured in a three-dimensional harmonic potential, the critical exciton number N c scales as N c ∝ T 3 ( N c ∝ T 3/2 in free space). Therefore, the optical power required to reach the critical exciton number in a harmonic trap is proportional to T 6 , whereas the specific heat of semiconductors scales as T 3 . This naive consideration indicates that the lower the exciton temperature is, the more favourable the conditions are for achieving BEC with the least lattice temperature increase. High-density excitation To increase the number of trapped paraexcitons while keeping the lattice temperature unchanged ( T L =354 mK), we chop the pump beam with appropriate duty cycles to make the average power constant (Methods). For ideal Bose particles well above the critical number, a large occupation number of the ground state is expected. 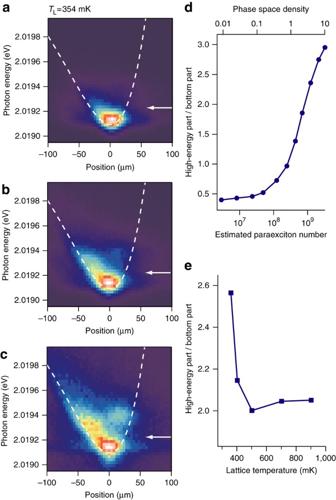Figure 3: Anomalous luminescence of 1sparaexcitons when crossing the phase boundary for Bose–Einstein condensation. Spatially resolved luminescence signals taken atTL=354 mK, where the estimated paraexciton numberNin the trap is (a) 2×107(b) 5×108and (c) 2×109. Signal intensities are normalized. Arrows show the boundary of the higher-energy (2.01924–2.02004 eV) and bottom (2.01902–2.01921 eV) parts of the signal. (d) Ratio between the higher-energy and bottom parts of the signal versus the estimated paraexciton number. Phase space density is calculated from the estimated number and the volume of the cloud at exciton temperatureT=0.8 K, assuming ideal, non-interacting bosons. (e) The ratio versus the lattice temperature under a constant excitation density (N=2×109at 354 mK). Instead, as shown in Figure 3 , we have observed anomalous spectra when the paraexciton number crosses the critical number. With increasing estimated paraexciton number, N =2×10 7 , 5×10 8 and 2×10 9 ( Fig. 3a–c , respectively), a high-energy signal appears suddenly up to around 400 μeV above the potential minima. In Figure 3d , we plot the integrated emission intensity ratio between the higher-energy part (2.01924–2.02004 eV) and the bottom part (2.01902–2.01921 eV) versus the paraexciton number. A threshold-like rise of the ratio near N c at an exciton temperature of 0.8 K is apparent, indicating that the BEC transition occurs at the condition expected for ideal bosons. We also examine the temperature dependence measurements under a constant excitation density. We set the excitation level at the maximum density of ( Fig. 3d ) N =2×10 9 at T L =354 mK. The lattice temperature dependence of the ratio also shows an abrupt increase at T L ∼ 400 mK ( Fig. 3e ), demonstrating the BEC transition of excitons (lowering T L results in a slight exciton temperature drop and an increased exciton number). In estimating N , we first calculated N in the weakest excitation linear regime from the amount of optical absorption (36% of incident power on the refrigerator) and the lifetime of paraexcitons, assuming an overall trap collection efficiency of 30%. The validity of this method of exciton counting has been confirmed by exciton Lyman spectroscopy [16] . Using the data from this low-density regime, we determined N for higher-density excitations by comparing the emission signal intensity of the bottom part. This prevents possible ambiguity in estimating the number of paraexcitons, although rate equations taking into account the inelastic collision-induced loss (therefore effectively shorter lifetime in high-density regions) estimates the similar number (see also Supplementary Information ). Figure 3: Anomalous luminescence of 1 s paraexcitons when crossing the phase boundary for Bose–Einstein condensation. Spatially resolved luminescence signals taken at T L =354 mK, where the estimated paraexciton number N in the trap is ( a ) 2×10 7 ( b ) 5×10 8 and ( c ) 2×10 9 . Signal intensities are normalized. Arrows show the boundary of the higher-energy (2.01924–2.02004 eV) and bottom (2.01902–2.01921 eV) parts of the signal. ( d ) Ratio between the higher-energy and bottom parts of the signal versus the estimated paraexciton number. Phase space density is calculated from the estimated number and the volume of the cloud at exciton temperature T =0.8 K, assuming ideal, non-interacting bosons. ( e ) The ratio versus the lattice temperature under a constant excitation density ( N =2×10 9 at 354 mK). Full size image As mentioned above, in this case inelastic collision is essential for inducing the anomalous spatial spectral profiles of the signal. Therefore, we exclude the effect of the renormalized energy due to the mean-field shift associated with the elastic scattering of the condensate [26] . We propose a feasible scenario: competition between bosonic-stimulated scattering and inelastic scattering-induced loss in the condensate. Considering the inelastic scattering cross-section (or collisional loss coefficient on the order of 10 −16 cm 3 ns −1 ) and the spatial spread of the ground-state wavefunction of 1.4 μm at full width at half maximum, the ground state is apparently unstable against ∼ 10 9 condensed paraexcitons. This yields a collision-induced lifetime of less than 100 fs. By analysing rate equations considering collisional loss in the condensate and its redistribution to the thermal part, we estimate that the maximum condensate fraction is around 1% (80% in the case of ideal bosons) with a bosonic-stimulated scattering rate of 7 ns −1 . Paraexcitons expelled from the condensate explains the enhancement of the observed signal in the high-energy part ( Supplemenary Information ). This situation is analogous to several examples of atomic condensates. It is well known that the condensate fraction for atomic hydrogen is limited to several percent due to the small s -wave elastic scattering length and two-body collisional loss [4] . It is indeed predicted that the spatial compression of the condensate in a magnetic trap leads to an enhanced relaxation due to the two-body (dipolar) scattering, and that the increase in the released hot atoms can be a measure of the transition to BEC [27] . This 'relaxation explosion' is exactly the case for the current system where the elastic scattering length is comparably small and the two-body collision-induced loss is present. Therefore, we conclude that dilute excitons obey the Bose–Einstein statistics and form BEC when the system crosses the phase boundary for ideal bosons, although depicting the precise phase diagram requires further experimental efforts. For excitons in semiconductors, in addition, the efficient cooling of the paraexcitons having high translational momenta via emission of acoustic phonons has an important role to thermalize the exciton gas and to force expelled excitons to come back towards the bottom of the trap (see also our numerical simulation in Supplementary Information ). For 7 Li atoms with attractive interactions, the three-body loss leads to the collapse of BEC. The observed condensate fraction is a few percent at most, as determined by the attractive forces and the repulsion due to position-momentum uncertainty [3] , [28] . To prepare a large condensate fraction, we must reduce the local density below 10 15 cm −3 . Therefore, making colder exciton gas is essential. Active methods to enhance exciton–phonon coupling, together with better sample quality, are desired. A dynamic trap can be helpful for making a shallower trap potential upon growth of the condensate. Because inelastic scattering dominates elastic scattering, evaporative cooling does not work in this system. Elucidating the mechanism for the large inelastic scattering cross-section is apparently crucial. It is interesting to compare our results with recently observed ultracold chemical reactions of molecules [29] and rapid inelastic collision of quantum-degenerate p -wave molecules [30] . Sample cooling A cryogen-free 3 He refrigerator (Oxford Instruments, Heliox-ACV) was used to cool the high-purity Cu 2 O single-crystal conductively. The size of the optical windows and the numerical aperture were carefully chosen to prevent any heat load into the coldest plate of the refrigerator. The lowest crystal temperature without irradiation of the excitation beam was 278 mK. The sample was 5.3×5.3×9.1 mm in size. Stress was applied along the [100] axis of the crystal by pressing the crystal with a lens and a built-in spring. Weak luminescence light from the trapped paraexciton gas was collected from the (110) surface. Generation of excitons The excitation laser was a cw ring dye laser at 606 nm (Coherent, 899-21). For an incident optical power of more than 250 μW, the excitation beam was chopped using an acousto-optic modulator and a high-isolation switch and was coupled into a single-mode optical fibre to reduce scattered light. We thereby obtained a high on-off extinction ratio of 2×10 7 . The repetition rate was 500 Hz. We set the duty cycle D cycle when increasing the 'on' power P on of the quasi-cw excitation light, so that the average power is constant. However, at high excitation intensity, the paraexciton number increases only sublinearly. This results in a small-integrated luminescence intensity because the duty cycle is reduced. In such cases, a high extinction ratio is essential because weak residual light in the 'off' time results in a considerable amount of signal under weak excitation. Spatially resolved luminescence The magnified (×4) luminescence image of the trapped exciton gas was collected (numerical aperture 0.07) and dispersed by a 50-cm spectrometer. An EMCCD camera (Andor, DU970N-BV) detected the time-integrated signal. The integration time ranged from 100 to 1,500 s. The entrance slit of the spectrometer, which was parallel to the z -axis, captured only the central 7.5 μm (30 μm in the magnified image) of the gas. The vibration (amplitude ∼ 10 μm) of the sample was actively cancelled using a pair of piezoelectric transducers (PZTs) in the imaging section of the setup by monitoring the displacement using a laser diode and a position-sensitive photodetector (the spatial resolution was 0.76 μm). The signal intensity of the Γ 5 − -phonon-assisted luminescence of paraexcitons was comparable to the detection noise level in our allowable integration time. How to cite this article: Yoshioka, K. et al . Transition to a Bose–Einstein condensate and relaxation explosion of excitons at sub-Kelvin temperatures. Nat. Commun. 2:328 doi: 10.1038/ncomms1335 (2011).